Nanoarchitectured materials composed of fullerene-like spheroids and disordered graphene layers with tunable mechanical properties Type-II glass-like carbon is a widely used material with a unique combination of properties including low density, high strength, extreme impermeability to gas and liquid and resistance to chemical corrosion. It can be considered as a carbon-based nanoarchitectured material, consisting of a disordered multilayer graphene matrix encasing numerous randomly distributed nanosized fullerene-like spheroids. Here we show that under both hydrostatic compression and triaxial deformation, this high-strength material is highly compressible and exhibits a superelastic ability to recover from large strains. Under hydrostatic compression, bulk, shear and Young’s moduli decrease anomalously with pressure, reaching minima around 1–2 GPa, where Poisson’s ratio approaches zero, and then revert to normal behaviour with positive pressure dependences. Controlling the concentration, size and shape of fullerene-like spheroids with tailored topological connectivity to graphene layers is expected to yield exceptional and tunable mechanical properties, similar to mechanical metamaterials, with potentially wide applications. Carbon materials are known to possess strong chemical bonds with sp , sp 2 and sp 3 hybridizations, displaying an impressively rich variety of atomic arrangements, such as graphene, fullerenes, nanotubes and so on, in addition to the well-known crystalline forms of graphite and diamond. Distinct mechanical behaviours of various carbon materials originate from the difference in these atomic structures. One of the unique features of sp 2 hybridization in graphene layers is the high in-plane rigidity and out-of-plane flexibility, capable of resisting in-plane stretching and compression while sustaining large elastic distortion through bending and folding. Rolled-up graphene sheets are the basic structural elements in fullerenes and nanotubes. Under pressure, the circular cross-section of the nanotubes can undergo various reversible changes to become polygon-, oval-, racetrack- and peanut-like [1] . Given the structural flexibility and high in-plane strength, some sp 2 carbon forms, such as aligned carbon nanotube films and three-dimensional (3D) interconnected graphene foams with micron-scaled open-air porosity as a structural variable [2] , [3] , [4] , display certain mechanical characteristics similar to those of architectured materials, especially metamaterials. Mechanical metamaterials are a special type of architectured material composed of tailored functional building blocks periodically arranged and connected to yield unusual mechanical properties, such as negative Poisson’s ratio, negative compressibility and negative incremental stiffness, all of which are not common in natural materials [5] , [6] , [7] . The metamaterials gain their exceptional properties not only from their composition but also from their exactingly designed architectures with special shape, geometry, size, orientation and arrangement. Because of the skeletal nature of the architecture, metamaterials generally have the advantage of being extremely lightweight [8] . The length scales of these periodical building blocks (similar to unit cells in crystalline materials) are typically on the order of tens of microns and above, thereby precise fabrication techniques (for example, lithography) are commonly needed [7] , limiting their assemblies to relatively large scales (centimetres and above). Therefore, it is more practical and cost-effective to produce statistically averaged fine-scaled building blocks, for example, as shown by some carbon and polymer foams [3] , [4] , [5] , [9] . A combination of different sp 2 carbon forms may add more variations of architectural building blocks to fine-scaled mechanical metamaterials, although designing and producing nanometre-scaled building blocks remain a technical challenge. Glass-like carbon (GC), a class of nongraphitizing carbon made by firing polymeric precursors such as phenolic resin or furfuryl alcohol resin in an inert atmosphere, possesses a number of advantageous properties including low density, high hardness and strength, high impermeability to both gases and liquids, high temperature stability and extreme resistance to chemical corrosion [10] . These properties are essential for the application of GC to engineering components under extreme environmental conditions. GC has been extensively investigated recently because of its fascinating high-pressure behaviours [11] , [12] , [13] , [14] . A fully sp 3 -bonded amorphous carbon with diamond-like strength was reversibly transformed from cold compressing type-I GC above 40 GPa (ref. 11 ). Nanocrystalline diamonds were produced by direct conversion of GC above 15 GPa and 1,600 °C (ref. 15 ). The structure of GC has been long debated [16] , [17] , but is now generally accepted to consist of nearly 100% sp 2 bonding. Type-I GC, which is produced at temperatures <2,000 °C, consists mainly of randomly distributed curved graphene layer fragments [10] , [18] . Type-II GC, fabricated at higher temperatures (~2,500 °C), contains self-assembled fullerene-like spheroids (FLS) of nanometre sizes, dispersed within, and interconnected by, a 3D disordered multilayer graphene (DMLG) matrix [10] , [18] , [19] . The structure of DMLG is similar to that of type-I GC [10] , [18] , [19] . Thus, type-II GC can be envisaged as FLSs encased in disordered graphene layers possessing a Swiss-cheese like nanostructure ( Fig. 1 ), which has a number of similarities to mechanical metamaterials [20] , but with statistical characteristic building blocks (that is, FLS) at nanometre scales. Thus, it is expected that type-II GC may inherit distinct properties of individual allotropes and possess exceptional elastic and mechanical properties. 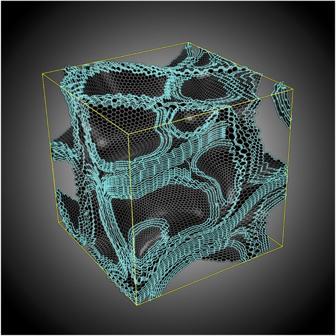Figure 1: FLS encased in a disordered multilayer graphene matrix. The structure can be viewed as a Swiss-cheese like nanostructure. Typical sizes of the FLS are ~5–10 nm. Figure 1: FLS encased in a disordered multilayer graphene matrix. The structure can be viewed as a Swiss-cheese like nanostructure. Typical sizes of the FLS are ~5–10 nm. Full size image Here we investigate the structure–property relationship of the GC under compression. Hydrostatic compression behaviour and elastic moduli are measured using in situ techniques of direct volume determination and acoustic wave velocity, respectively. The results of volume compression from both methods agree well with each other. Structural response to pressure is studied by in situ synchrotron X-ray diffraction. Axial stress–strain relations under various controlled confining pressures are established by triaxial deformation experiments. On the basis of the structure of type-II GC ( Fig. 1 ), with the aid of molecular dynamics (MD) simulations, an atomistic model is proposed to explain the unusual, and pressure-tunable, compression and elastic properties of type-II GC. This points to potential routes for developing new carbon-based nanoarchitectured materials with a unique combination of desired properties such as high compressibility, superelasticity, high toughness and zero/negative Poisson’s ratio, in addition to other known attractive properties. High compressibility and recovery Under hydrostatic pressure, type-I GC compresses smoothly, showing a compressibility higher than that of C 60 (ref. 21 ; Fig. 2a ). Type-II GC exhibits even higher compressibility than that of type-I GC. A cusp is clearly observed in the compression curve of type-II GC around 2 GPa, where compressibility displays a sudden jump with increasing pressure (inset of Fig. 2a ). Despite this abnormal behaviour, the compression is reversible up to ~11 GPa (corresponding to ~40% volume reduction), beyond which permanent volume reduction is observed. Samples recovered from compression to 35.5 GPa show a roughly 10% permanent densification ( Supplementary Fig. 1 ), suggesting that some FLS have collapsed. 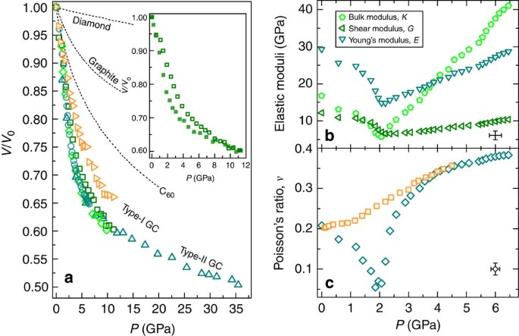Figure 2: Compression data and elastic moduli of type-II GC. (a) Compression curves obtained by optical imaging and acoustic measurements. Up-pointing triangles: compression to 35.5 GPa in helium pressure medium; diamonds: to 9.8 GPa in methanol–ethanol (4:1); squares: to 11.2 GPa in helium pressure medium; circles: compression data from acoustic measurements showing consistent results with those from the digital imaging method (triangles, diamonds and squares). Compression of type-I GC in methanol–ethanol (4:1) as a pressure-transmitting medium to 11.2 GPa (right-pointing triangles) is also shown for comparison. Dashed lines are compression curves of diamond57, graphite58and C60(ref.21), for comparison. The inset inais an enlarged view of type-II GC compression (open squares) and decompression (solid squares) to a pressure of 11.2 GPa. (b) Elastic moduli of type-II GC determined from acoustic wave velocity measurements to 6.5 GPa. (c) Poisson’s ratio of type-II GC (diamonds), calculated from elastic moduli shown inb, as a function of pressure. Poisson’s ratio of type-I GC (squares) is also shown for comparison. Errors in pressure in the diamond anvil cell and Paris-Edinburgh cell experiments are less than 0.10GPa and 0.15GPa, respectively. Errors in relative volume inaare the standard deviations in multiple imaging measurements. Errors in elastic moduli and Poisson's ratios are propagated from their relations with the elastic wave velocities and densities. Experimental errors inaare less than the size of the symbols. Typical error bars are shown inbandcat lower right corner. Figure 2: Compression data and elastic moduli of type-II GC. ( a ) Compression curves obtained by optical imaging and acoustic measurements. Up-pointing triangles: compression to 35.5 GPa in helium pressure medium; diamonds: to 9.8 GPa in methanol–ethanol (4:1); squares: to 11.2 GPa in helium pressure medium; circles: compression data from acoustic measurements showing consistent results with those from the digital imaging method (triangles, diamonds and squares). Compression of type-I GC in methanol–ethanol (4:1) as a pressure-transmitting medium to 11.2 GPa (right-pointing triangles) is also shown for comparison. Dashed lines are compression curves of diamond [57] , graphite [58] and C 60 (ref. 21 ), for comparison. The inset in a is an enlarged view of type-II GC compression (open squares) and decompression (solid squares) to a pressure of 11.2 GPa. ( b ) Elastic moduli of type-II GC determined from acoustic wave velocity measurements to 6.5 GPa. ( c ) Poisson’s ratio of type-II GC (diamonds), calculated from elastic moduli shown in b , as a function of pressure. Poisson’s ratio of type-I GC (squares) is also shown for comparison. Errors in pressure in the diamond anvil cell and Paris-Edinburgh cell experiments are less than 0.10GPa and 0.15GPa, respectively. Errors in relative volume in a are the standard deviations in multiple imaging measurements. Errors in elastic moduli and Poisson's ratios are propagated from their relations with the elastic wave velocities and densities. Experimental errors in a are less than the size of the symbols. Typical error bars are shown in b and c at lower right corner. Full size image Anomalous elastic moduli and nearly-zero Poisson’s ratio We measured longitudinal and shear wave velocities simultaneously on type-I and -II GC up to 6.5 GPa ( Supplementary Figs 2 and 3 ). Density ( ρ ) under pressure was obtained by integrating bulk sound speed ( V B ) by assuming that the sample remained isotropic throughout compression [22] , [23] . With the density data, bulk ( K ), shear ( G ) and Young’s ( E ) moduli are derived from sound velocities ( Supplementary Figs 2 and 3 ). Figure 2b displays the moduli of type-II GC as a function of pressure. All moduli decrease abnormally with increasing pressure up to 2 GPa, where a sharp reversal to positive pressure dependence is observed. The change is rather dramatic: K, G and E are reduced, respectively, by 34%, 58% and 51% of the ambient pressure values at ~2 GPa, and then they increase linearly up to 6.5 GPa. The corresponding pressure derivatives K ′, G ′ and E ′, obtained by linear fits to the moduli with pressure, are 7.98, 0.99 and 3.19, respectively, above 2 GPa. The large jump in K ′, from negative below 2 GPa to about twice the normal value of ~4, is striking. Figure 2c shows Poisson’s ratio ( ν ) calculated according to the relation ν =(3K−2G)/(6K+2G). Upon compression, ν decreases from 0.2 to near zero (0.05) at 2 GPa, where it turns sharply and rises rapidly. Within a narrow pressure interval (from 2 to 3 GPa), ν jumps to 0.3. In comparison, the Poisson’s ratio of type-I GC does not show such turn-over and exhibits positive pressure dependences from 0.2 at ambient pressure to 0.36 at 4.5 GPa ( Fig. 2c ). Superelastic behaviour GC is known to be brittle under ambient pressure [24] . However, deformation behaviour of type-II GC reported previously based on indentation tests shows a remarkable recovery of indentation impressions with loads up to ~100 N and significantly nonlinear stress–strain relations with large stress–strain hysteresis loops [24] , [25] . Our triaxial deformation experiments on cylindrical samples ( Fig. 3 and Supplementary Fig. 4 ), in contrast, show that the differential stress versus axial strain relation for type-II GC is largely linear and recoverable up to unusually high strains ( ca 6%). Axial deformation experiments under low confining pressures (10–30 MPa) show that type-II GC deforms linearly and recoverably up to ~4% axial strain without a clear sign of yielding ( Fig. 3a ). Beyond 4% strain, the samples failed by brittle fracturing. In the Griggs apparatus, at 0.5 GPa confining pressure ( Fig. 3b and Supplementary Fig. 4 ), the linear relationship continues up to ~6% strain, beyond which the material yields. With further increasing confining pressure, the material yields at progressively lower strains, but is still above 4%. 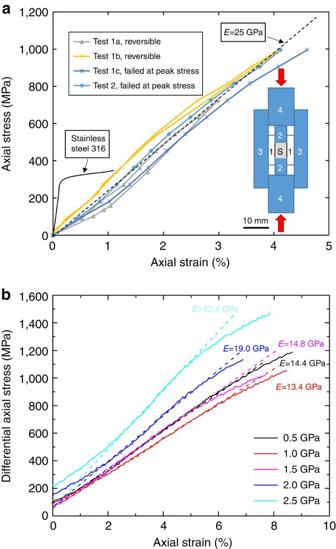Figure 3: Triaxial tests of type-II GC. (a) Under low confining pressure. Inset shows the experimental set-up. S, sample; 1, Teflon (PTFE) sleeve; 2, inner tungsten carbide (WC) pistons; 3, WC confining sleeve; 4, outer WC pistons. Red arrows indicate the loading direction. The confining pressure was controlled by the strength of Teflon at around 10–30 MPa (ref.55). Typical errors are estimated to be ±0.2% in axial strain and ±20 MPa in axial stress. Curves for testsFig. 1a, b, and care from one rod sample. In all cases, no yielding was detected before failure, within rather large uncertainties. Black dashed straight line is the expected linear elastic response of a material with Young’s modulus of 25 GPa, which is approximately the value determined from acoustic wave velocity measurements for type-II GC rod at hydrostatic 50 MPa (Supplementary Fig. 7). Black solid curve corresponds to room temperature stress–strain curve of stainless steel 316 during axial extension deformation28. Under this confining pressure, type-II GC is linearly superelastic up to 4% strain and it can sustain up to 1 GPa axial stress. For comparison, stainless steels are seven to eight times stiffer in Young’s modulus than type-II GC, but they yield at much lower strains (typically ~0.2%), with much lower yield strength (0.3 GPa). (b) Differential stress–axial strain curves of type-II GC rods at various confining pressures from 0.5 to 2.5 GPa. The linear portions (indicated by the dashed lines) are elastic, with the slopes corresponding to the Young’s moduli at various pressures. Similar to the ultrasonic measurements (Supplementary Fig. 7), a minimum in E was found in this case at 1.0 GPa. At pressures, the samples remained elastic up to 6% strain (at 0.5 GPa), above which yielding is observed with high-pressure curves showing greater nonlinearity. Nonlinearity at low stresses is because of issues discussed above (see Methods). The recovered samples showed ~2% permanent shortening with no sign of fracturing. Figure 3: Triaxial tests of type-II GC. ( a ) Under low confining pressure. Inset shows the experimental set-up. S, sample; 1, Teflon (PTFE) sleeve; 2, inner tungsten carbide (WC) pistons; 3, WC confining sleeve; 4, outer WC pistons. Red arrows indicate the loading direction. The confining pressure was controlled by the strength of Teflon at around 10–30 MPa (ref. 55 ). Typical errors are estimated to be ±0.2% in axial strain and ±20 MPa in axial stress. Curves for tests Fig. 1a, b, and c are from one rod sample. In all cases, no yielding was detected before failure, within rather large uncertainties. Black dashed straight line is the expected linear elastic response of a material with Young’s modulus of 25 GPa, which is approximately the value determined from acoustic wave velocity measurements for type-II GC rod at hydrostatic 50 MPa ( Supplementary Fig. 7 ). Black solid curve corresponds to room temperature stress–strain curve of stainless steel 316 during axial extension deformation [28] . Under this confining pressure, type-II GC is linearly superelastic up to 4% strain and it can sustain up to 1 GPa axial stress. For comparison, stainless steels are seven to eight times stiffer in Young’s modulus than type-II GC, but they yield at much lower strains (typically ~0.2%), with much lower yield strength (0.3 GPa). ( b ) Differential stress–axial strain curves of type-II GC rods at various confining pressures from 0.5 to 2.5 GPa. The linear portions (indicated by the dashed lines) are elastic, with the slopes corresponding to the Young’s moduli at various pressures. Similar to the ultrasonic measurements ( Supplementary Fig. 7 ), a minimum in E was found in this case at 1.0 GPa. At pressures, the samples remained elastic up to 6% strain (at 0.5 GPa), above which yielding is observed with high-pressure curves showing greater nonlinearity. Nonlinearity at low stresses is because of issues discussed above (see Methods). The recovered samples showed ~2% permanent shortening with no sign of fracturing. Full size image The linear stress–strain relation contrasts what is reported on the basis of indentation experiments [24] , [25] . The discrepancy is attributed to the fact that indentation experiments are nonisobaric and both stress and strain vary spatially in the sample. In our triaxial deformation measurements, slopes of the stress–strain curves are consistent with Young’s moduli determined by our ultrasonic measurement at similar confining pressures; thus, the deviation from linearity indeed signifies yielding ( Fig. 3b ). The large linear elastic strain rivals the maximum strain (8%) of shape-memory materials such as NiTi alloys and zirconia ceramics [26] , [27] . Furthermore, although the material is elastically ‘soft’ (highly compressible), it has an ultrahigh strength over 1 GPa because of the remarkably wide elastic regime. For comparison, stainless steel, with Young’s modulus —approximately seven to eight times that of type-II GC, yields at linear strains of ~0.2%, with strengths only on the order of 0.3 GPa (ref. 28 ). Structural change in the DMLG matrix of type-II GC Structure factors of types-I and -II GC, determined from X-ray diffraction, are remarkably similar ( Fig. 4 ), suggesting that the main structural elements in both types of GC are DMLGs. Both structures are dominated by intense peaks at ~1.9, ~3.1 and ~5.3 Å −1 in the momentum transfer ( Q ) space, corresponding to interplanar spacings of ~3.3, ~2.0 and ~1.2 Å, in broad agreement with the (002), (100)/(101) and (110)/(112) d -spacings of graphite. These peaks, significantly broader than crystalline graphite, are similar to those observed in the disordered carbon phase produced by compressing C 60 to high pressures [29] . The weak peaks around 3.8 and 6.2 Å −1 are high order diffractions of the first two strong peaks. No obvious features from FLS are present in the diffraction patterns, indicating their random spatial distribution and irregular size distribution. The pair distribution functions G( r ) of type-II GC at ambient pressure ( Fig. 4d ) show the first peak at 1.36(1) Å, which reflects the first neighbour distance and is shorter than 1.42 Å of graphite. The second peak in G( r ) at 2.46(1) Å, representing the average distance of the shortest diagonal in the carbon hexagon ring (second neighbour), is close to the diagonal distance of 2.47 Å in graphite. 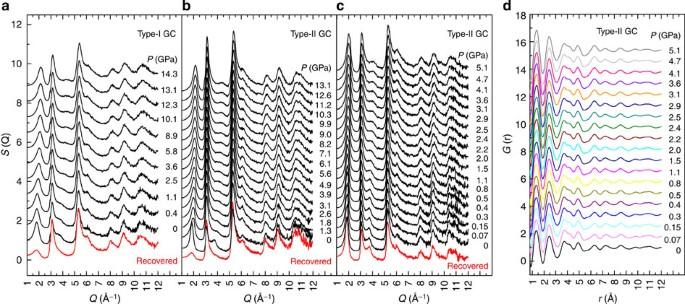Figure 4: Structure factorsS(Q) and pair distribution functionsG(r) of types-I and -II GC. (a)S(Q) of type-I GC to 14.3 GPa (black solid curves shifted in the vertical axis for clarity). TheS(Q) of the recovered sample from 14.3 GPa (red curve) is plotted for comparison. (b,c)S(Q) of type-II GC to 5.1 and 13.1 GPa (black solid curves), respectively. Structure factors of the recovered samples from 13.1 and 5.1 GPa (red curves) are plotted inb,c, respectively, for comparison. Note that theS(Q) of the recovered sample from 5.1 GPa is almost identical to that from the sample before compression. (d)G(r) of type-II GC to 5.1 GPa derived fromS(Q) data inc. The scales ofS(Q) for the recovered samples andG(r) at ambient pressure are the actual sizes, and other data are shifted by 0.8 ina,d, and 0.5 inb,c, respectively, for clarity. Figure 4: Structure factors S (Q) and pair distribution functions G (r) of types-I and -II GC. ( a ) S (Q) of type-I GC to 14.3 GPa (black solid curves shifted in the vertical axis for clarity). The S (Q) of the recovered sample from 14.3 GPa (red curve) is plotted for comparison. ( b , c ) S (Q) of type-II GC to 5.1 and 13.1 GPa (black solid curves), respectively. Structure factors of the recovered samples from 13.1 and 5.1 GPa (red curves) are plotted in b , c , respectively, for comparison. Note that the S (Q) of the recovered sample from 5.1 GPa is almost identical to that from the sample before compression. ( d ) G (r) of type-II GC to 5.1 GPa derived from S (Q) data in c . The scales of S (Q) for the recovered samples and G (r) at ambient pressure are the actual sizes, and other data are shifted by 0.8 in a , d , and 0.5 in b , c , respectively, for clarity. Full size image Pressure dependences of various characteristic distances of the DMLG matrix are summarized in Fig. 5 . Typical errors in pressure measurements are less than 0.15 GPa. On normalized plots ( Fig. 5c,d ), the pressure dependence of the interlayer distances for types-I and -II GC is close to each other within experimental errors. This is to be expected as the DMLG matrix in type-II GC is structurally similar to type-I GC. 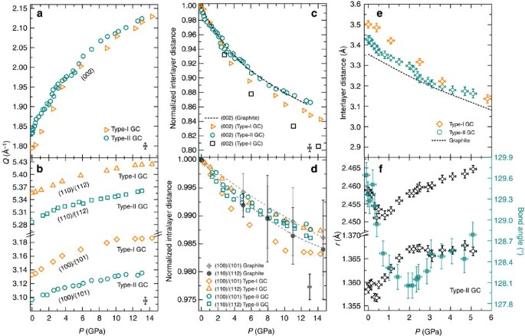Figure 5: Structural data of types-I and -II GC as a function of pressure. Because the interplanar spacings of GC are in broad agreement with the (002), (100)/(101) and (110)/(112)d-spacings of graphite, we use thed-spacing notation of graphite to represent the interlayer and intralayer distances of GC. (a) Interlayer distances analogous to (002) graphite. (b) Intralayer distances similar to (100)/(101) and (110)/(112) graphite. (c) Normalized interlayer distances. Open squares are data on type-I GC by ref.11. (d) Normalized distances similar to graphite (100)/(101) and (110)/(112). Solid grey diamonds and dashed curves of graphite intralayer distances are calculated from ref.59. From these data, volume compression of DMLG was evaluated. Note that the DMLG component of type-II GC appears slightly less compressible than type-I GC. (e) Interlayer distances derived from the first diffraction peak positions as a function of pressure (similar to graphite-(002)). The corresponding interlayer distances of graphite59are plotted as a dashed line for comparison. (f) Average first- (open circles) and second-neighbour (open diamonds) distances, derived from theG(r), as a function of pressure. The bond angles (solid squares) are derived from the ratio of the first- and second neighbour distances according to ref.30. The precisions are less than 0.002 Å for bond lengths and 0.2° for bond angles. Errors in pressure are typically less than 0.15 GPa. Errors in Q position are estimated from the standard deviations in fitting the first two peaks inFig. 4a, b and c. Errors inc,d,eare propagated from the uncertainties in Q. Errors infare derived from the standard deviations in fitting the first two peaks inFig. 4d. The current error bars (s.d.) are displayed at the lower right corner in (a–d) and plotted at the data in (e,f). Figure 5e shows actual interlayer distances of type-II GC as a function of pressure, as compared with that of type-I GC and graphite. Plotted in Fig. 5f is the average bonding angle, calculated according to ref. 30 , in the carbon ring as a function of pressure. The most prominent features of the bonding angle are the sharp decrease from 0 to 2 GPa and the rapid turn-around above. The total range of the bonding angle, 128° to ~130°, is significantly greater than the ideal bonding angle in carbon hexagon rings (120°). Figure 5: Structural data of types-I and -II GC as a function of pressure. Because the interplanar spacings of GC are in broad agreement with the (002), (100)/(101) and (110)/(112) d -spacings of graphite, we use the d -spacing notation of graphite to represent the interlayer and intralayer distances of GC. ( a ) Interlayer distances analogous to (002) graphite. ( b ) Intralayer distances similar to (100)/(101) and (110)/(112) graphite. ( c ) Normalized interlayer distances. Open squares are data on type-I GC by ref. 11 . ( d ) Normalized distances similar to graphite (100)/(101) and (110)/(112). Solid grey diamonds and dashed curves of graphite intralayer distances are calculated from ref. 59 . From these data, volume compression of DMLG was evaluated. Note that the DMLG component of type-II GC appears slightly less compressible than type-I GC. ( e ) Interlayer distances derived from the first diffraction peak positions as a function of pressure (similar to graphite-(002)). The corresponding interlayer distances of graphite [59] are plotted as a dashed line for comparison. ( f ) Average first- (open circles) and second-neighbour (open diamonds) distances, derived from the G (r), as a function of pressure. The bond angles (solid squares) are derived from the ratio of the first- and second neighbour distances according to ref. 30 . The precisions are less than 0.002 Å for bond lengths and 0.2° for bond angles. Errors in pressure are typically less than 0.15 GPa. Errors in Q position are estimated from the standard deviations in fitting the first two peaks in Fig. 4a, b and c . Errors in c , d , e are propagated from the uncertainties in Q. Errors in f are derived from the standard deviations in fitting the first two peaks in Fig. 4d . The current error bars (s.d.) are displayed at the lower right corner in ( a – d ) and plotted at the data in ( e , f ). Full size image Enormous volume reduction of FLS in type-II GC Because type-II GC can be viewed as DMLG matrix encasing FLS ( Fig. 1 ), the volume of type-II GC may be divided into two parts, V DMLG and V FLS . To the first approximation, we assume that FLS does not contribute to the mass of the sample, and that the DMLG component has a density close to that of graphite (2.25 g cm −3 ). Thus, the mass of the sample can be approximated as where subscripts 0 indicate ambient pressure (that is, 0.1 MPa). With the known density of type-II GC (1.42 g cm −3 ), we estimate the volumetric ratio of the two components as We further assume that, at any pressure P , the total volume reduction of the sample can be expressed by individual volumetric fractions ξ , that is, Our diffraction data show that DMLG behaves similarly to those of graphite and type-I GC ( Fig. 5c,d ). With the information of ξ GCII, P from our experiments ( Fig. 2a ), we obtain the compression behaviour of FLS. The results are shown in Fig. 6a . These spheroids, typically ~5–10 nm in linear dimension according to high-resolution transmission electron microscopy (HRTEM) observations ( Supplementary Fig. 5a ), appear to be extremely compressible. For a bulk sample compressed by 40% in volume (at ~11 GPa), the FLS component experienced an ~82% volume reduction. More remarkably, this enormous volume reduction is recoverable after pressure release (inset of Fig. 2a ). The overlap of structure factors between the starting material and the sample recovered from 5.1 GPa is consistent with the total recovery observed in volume measurements up to 11 GPa ( Figs 2a and 4c ). The HRTEM images on the sample recovered from 5.1 GPa reveal no major structural difference compared with the starting material ( Supplementary Fig. 5b ). The sample recovered from 13.1 GPa, on the other hand, shows minor differences in structure factors ( Fig. 4b ) and different microstructures from HRTEM ( Supplementary Fig. 5c ), indicating partial permanent collapse of FLS. 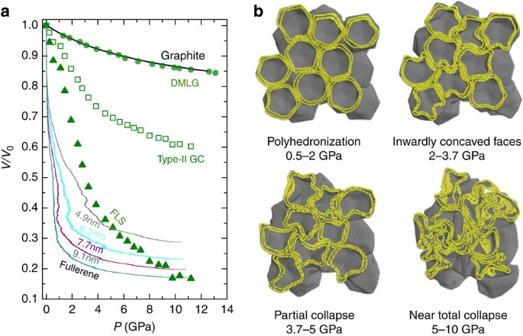Figure 6: Results of MD simulation on compression of fullerene arrays as compared with observed compression in type-II GC. (a) The volume compression of FLS (solid triangles) as derived from compression of DMLG observed by X-ray diffraction (solid circles) and total volume compression by direct sample volume measurements (open squares). Compression behaviour of graphite (black line)58is consistent with that of DMLG in type-II GC. Compression curves of MD simulated fullerene aggregates with sphere diameters 4.9, 6.3, 7.7 and 9.1 nm are plotted as solid lines. (b) Snapshots of fullerene aggregates with a sphere diameter of 4.9 nm at selected pressures from the MD simulations. Each inwardly deformed sphere is connected to a neighbouring outwardly protruding sphere, similar to the behaviour observed in mechanical metamaterials9,38, reducing the Poisson’s ratio (v) to zero. Figure 6: Results of MD simulation on compression of fullerene arrays as compared with observed compression in type-II GC. ( a ) The volume compression of FLS (solid triangles) as derived from compression of DMLG observed by X-ray diffraction (solid circles) and total volume compression by direct sample volume measurements (open squares). Compression behaviour of graphite (black line) [58] is consistent with that of DMLG in type-II GC. Compression curves of MD simulated fullerene aggregates with sphere diameters 4.9, 6.3, 7.7 and 9.1 nm are plotted as solid lines. ( b ) Snapshots of fullerene aggregates with a sphere diameter of 4.9 nm at selected pressures from the MD simulations. Each inwardly deformed sphere is connected to a neighbouring outwardly protruding sphere, similar to the behaviour observed in mechanical metamaterials [9] , [38] , reducing the Poisson’s ratio ( v ) to zero. Full size image MD simulations To better understand the role of FLS in the compression behaviour of type-II GC, we performed MD simulations on fullerene aggregates. For simplicity, all fullerenes are double-shell aggregates with outer sphere diameters from 1.4 to 14.7 nm. Each aggregate, containing ~300,000 carbon atoms, was assembled on the basis of a single fullerene size. Effects of the DMLG were ignored, as details of interaction between the DMLG and FLS components in type-II GC are still lacking. Our main goal for the MD simulation is to examine specifically the effects of FLS on the unique mechanical properties of type-II GC. The results are summarized in Fig. 6 and Supplementary Fig. 6 . Fullerene arrays with outer sphere diameters less than ~3 nm compress smoothly and elastically up to 10 GPa, consistent with experimental compression of C 60 molecular crystals [21] . For arrays with sphere diameters of 4.9–9.1 nm, compression curves exhibit a sudden jerk, which occurs at pressures from ~2 (for aggregate with 4.9-nm spheres) to ~0.5 GPa (9.1-nm spheres), because of partial collapse of the spheroids ( Supplementary Fig. 6 ). The pressure in which the jerk occurs is compared with the pressure of the cusp in the compression curve of type-II GC with fullerene diameters of ~5–10 nm ( Fig. 6a ). Figure 6b displays snapshots of the fullerene aggregates at selected pressures according to the MD simulations. With increasing pressure, the deformation of fullerene arrays may be categorized as the following four main stages: (1) spheres first become polyhedra with flattened faces; (2) some flattened faces concave inward; (3) upon further compression, some inwardly concave faces collapse, resulting in accelerated compression; (4) after compression to ~30%, the fullerene aggregates become more resistant to compression ( Fig. 6b ). Under pressure, type-II GC with FLS ranging from 5 to 10 nm in diameter exhibits much higher volume compressibility and greater elastic recovery ability than other known carbon materials, common metals and alloys, ceramics and even some organic polymers ( Figs 2a and 7 ). Under triaxial deformation, type-II GC exhibits both ultrahigh compressive strength (above 1 GPa) and superelasticity (recoverable linear strain up to 6%, comparable to, or even beyond, common shape-memory alloys and ceramics [26] , [27] ). To understand the remarkably high compressibility and superelastic behaviour of type-II GC, we need to examine the interaction of the structural components in GC. Two factors determine these unique properties: (a) average size and spatial distribution of the FLS, and (b) topological connectivity to the DMLG. While the former controls the compressibility of the material, interaction with the latter during deformation controls elastic moduli and Poisson’s ratio. 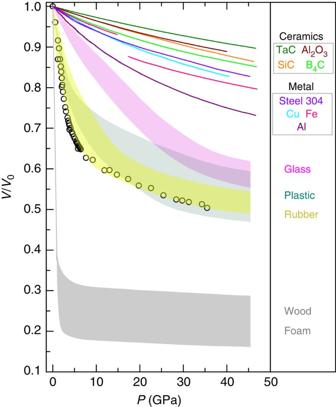Figure 7: Volume compression of various materials compared with type-II GC (black open circles). Materials included here are ceramics60,61,62,63, metals64,65,66,67, glasses (for example, high-density glass for nuclear pacific X-ray plate, Pyrex glass)64, plastics (for example, polyamide nylon, polyethylene, polyvinyl chloride and polycarbonate)64, rubbers (for example, silastic, neoprene and Goodrich D-402)64,68, wood (for example, pine and birch)64, porous carbon and polymer foams64. Type-II GC exhibits high-volume compressibility and elasticity, which rival those of soft organic polymers (for example, rubbers and plastics), but with remarkably high strength and hardness comparable to, or greater than, common metals and alloys (for example, steels, see the section on triaxial deformation tests above). Wood, carbon foams and polymer foams, on the other hand, are highly compressible (but nonrecoverable) at lower pressures because of the open porosities at large length scales, in contrast to the complete volume recovery of type-II GC up to 11 GPa (Fig. 2a). Figure 7: Volume compression of various materials compared with type-II GC (black open circles). Materials included here are ceramics [60] , [61] , [62] , [63] , metals [64] , [65] , [66] , [67] , glasses (for example, high-density glass for nuclear pacific X-ray plate, Pyrex glass) [64] , plastics (for example, polyamide nylon, polyethylene, polyvinyl chloride and polycarbonate) [64] , rubbers (for example, silastic, neoprene and Goodrich D-402) [64] , [68] , wood (for example, pine and birch) [64] , porous carbon and polymer foams [64] . Type-II GC exhibits high-volume compressibility and elasticity, which rival those of soft organic polymers (for example, rubbers and plastics), but with remarkably high strength and hardness comparable to, or greater than, common metals and alloys (for example, steels, see the section on triaxial deformation tests above). Wood, carbon foams and polymer foams, on the other hand, are highly compressible (but nonrecoverable) at lower pressures because of the open porosities at large length scales, in contrast to the complete volume recovery of type-II GC up to 11 GPa ( Fig. 2a ). Full size image The turn-over of the elastic moduli in type-II GC around 2 GPa ( Fig. 2b ) is an interesting anomalous phenomenon. In homogeneous materials, the diminishment of certain elastic moduli implies a structural transformation. Type-II GC, however, is not a homogeneously structured material at the atomic level. The observed X-ray characteristic distances reported in Figs 4 and 5 only reflect behaviour of the DMLG matrix, but not that of FLS. Dynamic interaction between DMLG and FLS must have played a critical role throughout compression. Our MD simulations on fullerene arrays offer a glimpse of the roles of FLS in the compression process. Type-II GC can be viewed as an architectured material consisting of nanosized FLS randomly dispersed in the DMLG matrix. The high compression of type-II GC is likely associated with the deformation of the fullerene spheroids, which have the ability to undergo large volume contraction as shown in Fig. 6a . Our MD simulations show that compression of fullerene arrays consists of four stages ( Fig. 6b ). This compression behaviour has certain similarity to that of carbon nanotubes, which has been extensively studied both experimentally and by simulations [1] , [31] , [32] , [33] . At pressures around 1.5–2.6 GPa, circular cross-sectioned nanotubes change into hexagonal or oval cross-sections with a decrease in bulk modulus revealed [31] , [33] . Upon further compression, carbon nanotubes undergo a series of reversible deformation from hexagonal or oval, to racetrack-like, and, finally, to peanut-like cross-sections [1] , [32] . The changes in cross-sections of deformed fullerene arrays ( Fig. 6b ) are more complex because of their original spherical shape. In the presence of the DMLG matrix, we thus expect FLS in type-II GC to deform in a way similar to re-entrance foams [9] . The C–C bond length of graphite, given by the nearest-neighbour distances, is 1.42 Å, and the C–C–C bond angle is 120°. The relatively short bond length and large bond angles in DMLG ( Fig. 5f ) suggest distortion of six-membered carbon rings and possible existence of seven- and eight-membered carbon rings. The overall decrease in bond angles in type-II GC up to 2 GPa suggests flattening of the originally bent graphene layers, while subsequent increase in the angle likely reflects large shear deformation in the carbon hexagon rings because of severe distortion and shrinking of the FLS. Similar turn-overs in elastic moduli have been observed in other glasses, such as SiO 2 glass [34] and polymerized silicate glasses [35] . The anomalous elastic behaviour is generally related to the gradual structural rearrangement, which leads to a more flexible material below the turn-over pressure point. The turn-over points have been found to have correlations with bond angles for SiO 2 glass [36] and polymerized silicate glasses [35] , [37] . Above the turn-over point, the changes in bond angles lead to a more homogeneous material. In contrast, depolymerized silicate glasses do not show such turn-over behaviour in elastic moduli. It has been pointed out that the lack of initial interstitial voids in depolymerized glasses plays an important role [35] . In this case, the anomalous behaviour of type-II GC is similar to those of SiO 2 glass and polymerized silicate glasses at a larger scale. A correlation between the elastic anomaly and the bond angle is also observed from the X-ray diffraction experiments ( Fig. 5f ). The encased FLS may be viewed as initial interstitial voids similar in polymerized glasses. We therefore interpret the elastic anomalous behaviour around 2 GPa as the gradual structural rearrangement involving deformation of interstitial voids (FLS) and rapid compression along weakly van der Waals bonded directions, followed by a homogenization process across the turn-over point. The homogenization process may also explain the observation of the great recovery of the bulk modulus above the turn-over point compared with the weak recovery of the shear modulus ( Fig. 2b ). The overall increasingly homogenized structure above 2 GPa results in the increase in bulk modulus, while large shear deformation still exists in the carbon hexagon rings because of the partial collapse of the FLS. The cross-sectional view of compressed fullerene aggregates at pressure shows significant deformation of the spheroids ( Fig. 6b ), forming inwardly concaved shapes similar to the re-entrant foams with negative Poisson’s ratio [5] , [9] . Each inwardly deforming side of a sphere is connected to a neighbouring outwardly protruding sphere, similar to that observed in macroscopic metamaterials [38] . It is such mutual constraints that result in rapidly decreasing Poisson’s ratio with pressure in type-II GC ( Fig. 2c ). Similarly, the mechanisms determining high compression, superelastic behaviour and recoverable ability are all coupled together. The superelastic behaviour is related to the highly compressible nature of fullerene spheroids and the recoverable ability because of the strong sp 2 bonding of the graphene layers. The high in-plane rigidity of sp 2 bonds is responsible for the high strength and recovery, and the out-plane flexibility is for the large elastic strain and determines the changes of fullerene geometry. The disordered graphene matrix has strong graphene planes towards all directions, thus endowing the high strength of the GC. The lack of orientated defects is also an important factor responsible for the superelastic behaviour. Significant progress has been made in recent years in producing hierarchical nanostructured carbon forms at various length scales [39] . The atomistic mechanism of deformation in type-II GC, along with the understandings from mechanical metamaterials, suggest that it is feasible to tailor mechanical properties of carbon-based nanoarchitectured materials by controlling the size, concentration and connectivity of the FLS, in addition to pressure tuning. For example, different batches of purchased type-II GC with similar density demonstrate some variations in the compressibility, elastic moduli and Poisson’s ratio under pressure ( Supplementary Fig. 7 ). In addition, the material can also be made with desired auxeticity at a desired pressure, by controlling the spatial distribution of the FLS. This would be a remarkable auxetic material: isotropic and homogeneous at nanometre scales, impermeable, lightweight, high hardness/strength, with the ability to withstand large deformation. Volumetric compression measured by digital imaging The types -I and -II GC plates and rods were from Alfa Aesar with ash values less than 100 p.p.m. The original GC plates had a size of 25 × 25 mm with a thickness of 4 mm, and the initial GC rods had a length of 50 mm with diameters of 2, 3, 4, 5 and 7 mm, respectively. The bulk densities were 1.54 (±0.03) g cm −3 for type-I GC, and 1.42 (±0.02) g cm −3 for type-II GC. Disks of types -I and -II GC, from the crushed GC plate, with thicknesses less than 20 μm were loaded into a rhenium gasket hole of 180 μm in diameter and 45-μm thick in a diamond anvil cell with anvils of 300-μm culet size. Helium or methanol–ethanol (4:1) mixture was used as the pressure-transmitting medium, depending on the maximum pressure desired. After gas-loading, sample chamber size decreased to a hole of ~120 μm in diameter. Pressure was measured using the ruby scale [40] . Digital images of the sample in the diamond anvil cell were recorded along the loading axis using a 3 Megapixel camera. This method can provide reliable compression information if the following conditions are met: [41] (a) the sample is completely imbedded in a truly hydrostatic medium; (b) the sample contracts isotropically under pressure; (c) the sample provides images with strong contrast relative to the medium; (d) and the sample is highly impermeable to the medium. We have loaded the GC samples ( Supplementary Fig. 1 ) in helium or methanol–ethanol (4:1) mixture, which provides a hydrostatic compression in the pressure range of this study (up to 12 GPa (ref. 42 )). For a glassy material, isotropical contraction under hydrostatic pressure is a reasonable assumption. The GC samples are opaque and provide strongly contrasting images under microscope. One unique feature of the type-II GC is its impermeability to gasses with a diffusion coefficient of 10 –9 cm 2 s −1 under ambient condition (from Alfa Aesar). The impermeability is comparable to crystalline Si and metals such as Al, Au and Ag (refs 43 , 44 ). Furthermore, the impermeability is verified by the consistent compression results when a different pressure medium (4:1 methanol–ethanol) was used. High-pressure acoustic velocity and density measurements Techniques of acoustic wave velocity measurements are given in refs 22 , 23 . The GC plate (or rod in Supplementary Fig. 7 ) was shaped into a cylindrical rod with a diameter of 2 or 2.5 mm and a length of ~0.6 mm used in acoustic measurement. Pressure transmission media include MgO and BN, and pressure was determined using the equation of state of MgO (ref. 45 ). The sample dimensions at high pressure were measured using the X-ray radiography technique with 1-μm resolution [22] . Together with the travel time information of acoustic signals from sample interfaces, we thus obtain the acoustic velocities. From the measured longitudinal ( V P ) and shear ( V s ) wave velocities, densities of the samples at pressures were deduced by assuming isotropic samples throughout the compression: where ρ P and ρ 0 are the densities of the samples at pressure P and ambient pressure P 0 , respectively; V B is the bulk sound velocity, γ = C P / C V ≈1 is the ratio of the specific heats at constant pressure and volume. For elastically isotropic materials, V B 2 = V P 2 −4 V S 2 /3. Acoustic velocities are converted to elastic constants on the basis of the following relations: bulk modulus K = ρ P ( V P 2 −4 V S 2 /3); shear modulus G = ρ P V S 2 ; Young’s modulus E = ρ P V S 2 (3 V P 2 −4 V S 2 )/( V P 2 − V S 2 ); Poisson’s ratio v =( V P 2 −2 V S 2 )/2( V P 2 − V S 2 ) or ν =(3 K –2 G )/(6 K +2 G ). High-pressure structural characterization In situ high-pressure X-ray diffraction of samples from the GC plate was carried out using the multiangle energy-dispersive technique in a Paris–Edinburgh cell installed at 16-BM-B beamline of HPCAT, at the Advanced Photon Source [22] , [23] . A Paris–Edinburgh cell was used with modified Drickamer–Toroidal-type anvils with a 4-mm-flat cup cell up to 14.3 GPa for type-I GC and 13.1 GPa for type-II GC. For type-II GC up to 5.1 GPa, a 12-mm-cup cell was used. The diffraction patterns were collected at multiple diffraction angles (2 θ : 3°, 4°, 5°, 7°, 9°, 11°, 14°, 18°, 23°, 29° and 35°). Collection time varied with diffraction angle, as intensities decreased with increasing angles. All patterns were collected until the maximum intensity reached at least 2,000 counts, to ensure reliable counting statistics. The structure factors S( Q ) and the pair distribution function G( r ) were deduced using the approach developed in refs 23 , 46 . Transmission electron microscopy measurements HRTEM measurements were performed on three type-II GC samples: a fresh starting material and samples recovered from 5.1 and 13.1 GPa, respectively. A JEOL 2010F(s) microscope was used to characterize the morphology of the samples. To prepare a TEM sample, a small piece of the type-II GC was crushed between two clean glass slides. The small particles were transferred on a copper TEM grid of 300 mesh with carbon-based lacey network support film. The TEM images were obtained at 200-kV operation voltages on sample particles located at open holes of the lacey support film on the grid, which ensures minimum background for high resolution. MD simulations Supercells containing ~300,000 carbon atoms, which form specific number of two-shell fullerene aggregates (nesting doll-like) with diameters between 0.7 and 14.7 nm, were generated and optimized at room temperature using MD calculations implemented in LAMMPS code [47] , and the atomic configurations were visualized by using the OVITO package [48] . Each fullerene molecular was icosahedral with 12 five-membered rings at each vertex position of the icosahedron, which was similar with the icosahedral-quasicrystal-like model of an onion carbon or BN particle [49] , [50] . In our computational scheme, isothermal–isobaric (NPT) ensemble and periodic boundary conditions were used. Tersoff potential was chosen to describe C–C bonding interactions [51] , which has been widely used for describing carbon materials such as amorphous carbon, carbon nanowires and carbon nanotubes [52] , [53] , [54] . Each supercell was first relaxed for 200 ps at ambient pressure and room temperature, and then compressed hydrostatically to a given pressure (1, 2, 4, 7 and 10 GPa) within 2 ns, and finally decompressed to ambient pressure within 2 ns. During the (de)compression process, the corresponding structure, volume and stress were recorded. The velocity of atomic movement resulting from the strain during (de)compression was less than 0.02 km s −1 , which was far less than the solid sound velocities. Therefore, the chosen timescale had little effect on the elastic deformation. Triaxial deformation tests Two types of triaxial deformation tests were conducted on type-II GC. For low confining pressures, a simple desk-top device was constructed as shown by the inset in Fig. 3 . Type-II GC rods with 5-mm diameter and 6.5–7 mm in length were surrounded by a polytetrafluoroethylene ([PTFE) (Teflon) sleeve inside a tungsten carbide (WC) ring. Double WC pistons were used to transmit axial load on the sample. The confining pressure was controlled by the strength of Teflon at ~10–30 MPa (ref. 55 ). Axial stress was determined on the basis of total load applied to the deformation pistons, with internal friction effects ignored. Axial strain was on the basis of total assembly length measurements, with deformation in the WC pistons ignored. Deformation experiments at higher pressures of 0.5, 1.0, 1.5, 2.0 and 2.5 GPa were conducted in a modified Griggs apparatus (for description and cell assembly, see ref. 56 ). The sample rod was 3 mm in diameter and 9.18 mm in length, surrounded by a Pb sleeve, which was served as the pressure medium during room temperature deformation. A Pb disc was placed on the top of the sample, to ensure quasi-hydrostatic loading before deformation. Once a desired pressure was reached, a deformation piston was advanced until it pressed on the sample. This ‘landing’ process was monitored by plotting the piston travel distance versus the differential stress recorded by the load cell. The ‘hit’ point was then defined by extending the linear portions of the stress-displacement curves before and after landing the piston on the sample (for example, the intersection of the two red dashed lines in Supplementary Fig. 4 ). This results in an uncertainty of strain measurements of about ±1% (or ~50–200 MPa in stress) before a 2% strain ( Fig. 3b ). In addition, because of friction effects of the solid media used in the Griggs apparatus and the out-flow (in-flow) of the Pb discs when advancing (retracting) of the piston was taking place, the stress-displacement curves exhibit nonlinearity at low stresses and large hysteresis loops when the piston reverses its direction. As a result, only shortening stress–strain curves could be reliably measured and true stress–strain behaviour can only be determined at stresses above ~200 MPa. How to cite this article: Zhao, Z. et al . Nanoarchitectured materials composed of fullerene-like spheroids and disordered graphene layers with tunable mechanical properties. Nat. Commun. 6:6212 doi: 10.1038/ncomms7212 (2015).